High-performance photocatalytic nonoxidative conversion of methane to ethane and hydrogen by heteroatoms-engineered TiO2 Nonoxidative coupling of methane (NOCM) is a highly important process to simultaneously produce multicarbons and hydrogen. Although oxide-based photocatalysis opens opportunities for NOCM at mild condition, it suffers from unsatisfying selectivity and durability, due to overoxidation of CH 4 with lattice oxygen. Here, we propose a heteroatom engineering strategy for highly active, selective and durable photocatalytic NOCM. Demonstrated by commonly used TiO 2 photocatalyst, construction of Pd–O 4 in surface reduces contribution of O sites to valence band, overcoming the limitations. In contrast to state of the art, 94.3% selectivity is achieved for C 2 H 6 production at 0.91 mmol g –1 h –1 along with stoichiometric H 2 production, approaching the level of thermocatalysis at relatively mild condition. As a benchmark, apparent quantum efficiency reaches 3.05% at 350 nm. Further elemental doping can elevate durability over 24 h by stabilizing lattice oxygen. This work provides new insights for high-performance photocatalytic NOCM by atomic engineering. Methane, the predominant constituent of natural gas, shale gas and combustible ice, has provoked increasing attention as an important feedstock for energy supply and chemical production [1] , [2] . Conventionally, direct conversion of CH 4 to value-added multicarbon (C 2+ ) compounds is achieved via thermocatalysis through nonoxidative or oxidative routes [3] , [4] , [5] . Nevertheless, undesired side reactions, such as carbon deposition in nonoxidative routes and CH 4 overoxidation in oxidative routes, inevitably occur in the thermochemical processes, concomitantly with insufficient selectivity and yield of C 2+ compounds. Meanwhile, high temperatures (700−1110 °C) and pressure (>1 MPa) are required for such thermocatalytic approaches, resulting in high energy consumption and capital input [6] , [7] . Under such circumstances, future development demands new approaches to direct methane conversion in mild condition. In this context, photocatalytic nonoxidative coupling of methane (NOCM), which requires only solar energy as energy input and CH 4 as a reactant, emerges as an appealing approach for the production of value-added C 2+ hydrocarbons and hydrogen [8] , [9] . Given strong oxidation capability and lattice oxygen reactivity, metal oxide photocatalysts have been mainly explored for photocatalytic NOCM [10] , [11] , [12] . Despite that, the use of metal oxide unavoidably results in unsatisfying photocatalytic NOCM selectivity and durability. In detail, the valence band of metal oxide is predominantly composed of O 2 p states [13] , [14] , enabling the photogenerated holes to concentrate on O sites for cleaving C–H bond of CH 4 . Once C–H bonds are cleaved, overoxidation of CH 4 would readily take place at the O sites while consuming lattice oxygen [15] , [16] . As an outcome, photocatalytic reactivity decays by losing lattice oxygen while overoxidation products, e.g., CO 2 and CO arise [17] , [18] , restricting the product selectivity and catalyst durability of the oxide-based photocatalytic NOCM. To overcome these limitations, the valence band of oxide photocatalysts should be rationally engineered. In the past decade, metallic single atoms (SAs) loaded nanostructures have attracted tremendous interest for photocatalysis [19] , one of whose advantages is their capability of tailoring photocatalyst electronic structure [20] . The incorporation of metallic d -orbital structure shows more occupied state in valence band maximum (VBM) and provides additional active sites in photocatalysts [21] , [22] . Against this background, we propose that tailoring VBM of oxide photocatalyst with metallic SAs could be a feasible approach to reduce the contribution of O 2 p states to valence band near-surface, suppressing the overoxidation of CH 4 with lattice oxygen. Here, taking TiO 2 , a widely used oxide photocatalyst as a proof-of-concept model, we report that incorporation of Pd SAs in oxide surface lattice can overcome the limitations upon screening a series of metallic SAs toward photocatalytic NOCM. According to the simulation of the material, the Pd–O 4 unit demonstrates the largest contribution to VBM of surface TiO 2 so as to accumulate photogenerated holes, which in turn dissociate C–H bonds at Pd SAs. Furthermore, the unique feature of Pd in stabilizing ∙CH 3 allows it to be the reaction site for coupling of reaction intermediates. As a result, the Pd SAs modified catalyst (Pd 1 /TiO 2 ) exhibits the highest performance toward C 2 H 6 production, with an apparent quantum efficiency of 3.05% at 350 nm and an extraordinary C 2 H 6 production rate of 0.91 mmol g –1 h –1 . More importantly, the occupied state of Pd–O 4 in VBM suppresses the overoxidation of CH 4 with lattice oxygen, which offers 94.3% selectivity toward C 2 H 6 production and substantially improved stability of oxide photocatalyst. Furthermore, a pertinent element (i.e., Si) is selected to dope the TiO 2 lattice for further stabilizing subsurface lattice oxygen to elevate catalyst durability over 24 h. Material screening and photocatalytic performance To screen metallic SAs with the largest contribution to VBM, we employ density functional theory (DFT) calculation to examine various SAs modified TiO 2 (M 1 /TiO 2 ) catalysts near the surface. The key to the reconstruction of VBM is the coordination of SAs with lattice oxygen. To this end, we select TiO 2 (001) plane as the surface for decorating metallic SAs because it contains relatively loosely packed oxygen atoms as illustrated in Fig. 1a , which allows the formation of the M–O bond between the metallic SAs and lattice oxygen of TiO 2 [23] . For metallic nanoparticles, such a bond structure can hardly be formed so that they are mainly loaded on the TiO 2 surface (Pd n /TiO 2 ). 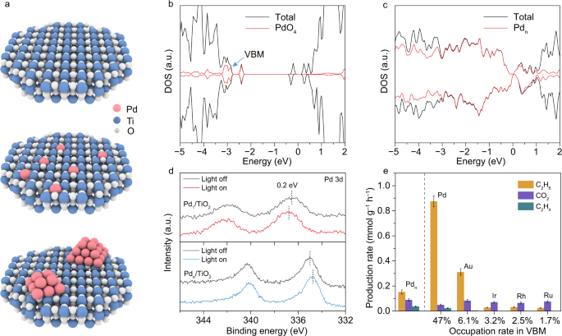Fig. 1: Screening of metallic SAs with large contributions to VBM of M1/TiO2for photocatalytic NOCM. aSchematic illustration for TiO2(001)-based models—pristine TiO2(top), Pd1/TiO2(middle), and Pdn/TiO2(bottom).b,cTotal density of states (TDOS) of Pd1/TiO2(b) and Pdn/TiO2(c). The red line represents the contribution of metals to TDOS, in which Pd–O4unit show the highest proportion in VBM (highlighted by blue arrow).dPd 3d XPS spectra of Pd1/TiO2and Pdn/TiO2under light irradiation indicating charge accumulation.eThe relationship of metal contribution in VBM and photocatalytic NOCM performance for various M1/TiO2as well as Pdn/TiO2. Reaction condition: 0.1 MPa CH4, 3 h light irradiation. The error bars represent the standard deviation of the experiments. Figure 1b, c shows the simulated density of states (DOS) for various M 1 /TiO 2 catalysts (see Supplementary Fig. 1 for other calculation results). For M 1 /TiO 2 catalysts, the composition of VBM is significantly altered although the decorated metallic SAs induce impurity states in the bandgap of TiO 2 . Pd–O 4 unit exhibits the largest contribution to VBM among all the studied catalysts, implying the potential of accumulating photogenerated holes. Notably, for the Pd nanoparticles, the photogenerated electrons would be concentrated at Pd due to the formation of Schottky junction (Fig. 1c ) [19] , [24] , while the photogenerated holes are remained in TiO 2 . Such an assumption is verified by Pd 3d X-ray photoelectron spectroscopy (XPS, Fig. 1d ). Specifically, under light irradiation, the binding energy for Pd 1 /TiO 2 is positively shifted for 0.2 eV, indicating the accumulation of photogenerated holes at Pd–O 4 unit. In contrast, Pd n /TiO 2 displays negatively shifted binding energy in Pd 3d XPS upon light irradiation (Supplementary Fig. 2 ). The charge accumulation is also proven by infrared spectroscopy with CO probe (Supplementary Fig. 3 ). Based on the theoretical simulation results, we prepare a series of metal SAs (Pd, Au, Rh, Ir, and Ru) modified TiO 2 for photocatalytic NOCM as shown in Fig. 1e . Generally, the TiO 2 loaded with Pd SAs, which owns the largest contribution to VBM of TiO 2 , demonstrates the highest activity and selectivity toward CH 4 −to−C 2 H 6 conversion. Moreover, computational and experimental results show that TiO 2 (001) is the optimal surface for loading Pd SAs as compared with other TiO 2 facets (Supplementary Fig. 4 ). Fig. 1: Screening of metallic SAs with large contributions to VBM of M 1 /TiO 2 for photocatalytic NOCM. a Schematic illustration for TiO 2 (001)-based models—pristine TiO 2 (top), Pd 1 /TiO 2 (middle), and Pd n /TiO 2 (bottom). b , c Total density of states (TDOS) of Pd 1 /TiO 2 ( b ) and Pd n /TiO 2 ( c ). The red line represents the contribution of metals to TDOS, in which Pd–O 4 unit show the highest proportion in VBM (highlighted by blue arrow). d Pd 3d XPS spectra of Pd 1 /TiO 2 and Pd n /TiO 2 under light irradiation indicating charge accumulation. e The relationship of metal contribution in VBM and photocatalytic NOCM performance for various M 1 /TiO 2 as well as Pd n /TiO 2 . Reaction condition: 0.1 MPa CH 4 , 3 h light irradiation. The error bars represent the standard deviation of the experiments. Full size image In this context, we focus on the investigation of the photocatalytic NOCM process on Pd 1 /TiO 2 in reference to pristine TiO 2 and Pd n /TiO 2 with similar Pd content (Supplementary Fig. 5 and Supplementary Table 1 ). Typically, all the samples are based on TiO 2 nanosheets dominated with (001) surface (Supplementary Figs. 6 and 7 ). To resolve the structure of Pd SAs, the Pd 1 /TiO 2 catalyst is examined by a series of microscopic and spectroscopic techniques. The high-angle annular dark-field scanning transmission electron microscopy (HAADF-STEM) images of Pd 1 /TiO 2 indicate that the Pd elements are atomically dispersed on the support (Fig. 2a and Supplementary Fig. 8 ), which is also verified by energy-dispersive X-ray spectroscopy (EDS) mapping (Fig. 2b ). To investigate the coordination environment of Pd in Pd 1 /TiO 2 catalyst, the catalyst is further characterized by synchrotron radiation-based X-ray absorption near-edge structure (XANES) spectroscopy (Supplementary Fig. 9 ). As revealed by extended X-ray adsorption fine structure (EXAFS) spectra in R space for Pd K-edge (Fig. 2c ), only a single peak for Pd–O coordination (1.53 Å) can be observed on Pd 1 /TiO 2 , confirming the domination of isolated Pd atoms in Pd 1 /TiO 2 catalyst. 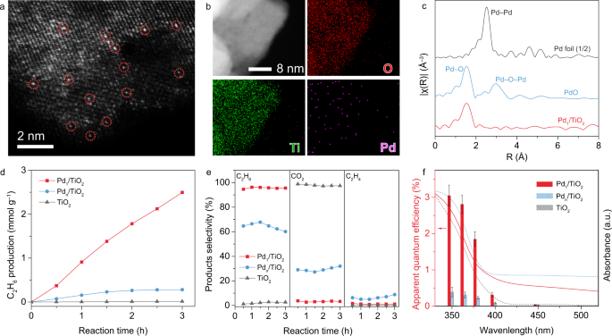Fig. 2: Structural characterization and photocatalytic NOCM performance of Pd1/TiO2catalyst. a–cSTEM image (a), elemental mappings (b) and Pd K-edge EXAFS spectra inRspace (c) of Pd1/TiO2. The isolated Pd atoms are marked with red circles in (a).d,eThe C2H6production rates (d) and the corresponding selectivity of C2H6, C2H4, and CO2(e) in 0.1 MPa CH4.fThe AQEs for CH4−to−C2H6conversion with their UV-vis diffuse reflectance spectra as references. The error bars represent the standard deviation of the experiments. According to the fitting, the average coordination number is determined to be 4 (Supplementary Table 2 ) [25] . The presence of isolated Pd atoms on the TiO 2 can be further affirmed via investigating the CO adsorption behavior on the catalysts (Supplementary Fig. 2 ) [26] , [27] . We thus conclude that the Pd atoms in Pd 1 /TiO 2 are isolated from each other and coordinated with four O atoms in TiO 2 to form Pd−O 4 units. Fig. 2: Structural characterization and photocatalytic NOCM performance of Pd 1 /TiO 2 catalyst. a – c STEM image ( a ), elemental mappings ( b ) and Pd K-edge EXAFS spectra in R space ( c ) of Pd 1 /TiO 2 . The isolated Pd atoms are marked with red circles in ( a ). d , e The C 2 H 6 production rates ( d ) and the corresponding selectivity of C 2 H 6 , C 2 H 4 , and CO 2 ( e ) in 0.1 MPa CH 4 . f The AQEs for CH 4 −to−C 2 H 6 conversion with their UV-vis diffuse reflectance spectra as references. The error bars represent the standard deviation of the experiments. Full size image Upon acquiring structural information for the catalyst, the detailed photocatalytic NOCM measurements are performed at room temperature under 600 mW cm –2 xenon arc lamp irradiation. As shown in Fig. 2d , pristine TiO 2 nanosheets exhibit a negligible C 2 H 6 production rate. This performance is due to the large contribution of O atoms to VBM, which leads to the direct participation of the lattice oxygen in CH 4 conversion. In detail, photogenerated holes in TiO 2 are predominantly concentrated at O atoms to cleave C−H bonds of CH 4 . As the activated methyl species can hardly desorb from O sites, they are vulnerable to overoxidation. As a result, CO 2 emerges as the major product with nearly 100% selectivity as shown in Fig. 2e . Since Pd nanoparticles play the role of electron accumulation, Pd n /TiO 2 does not suppress overoxidation to CO 2 but promotes C 2 H 6 production owing to dehydrogenation and stabilization of ∙CH 3 at Pd nanoparticles [28] , [29] . As such, Pd n /TiO 2 exhibits an initial rate of ~0.18 mmol g –1 h –1 for C 2 H 6 production in the first 1 h, which decreases gradually after 2 h of light irradiation due to lattice oxygen consumption by overoxidation (Fig. 2d ). The overoxidation is evidenced by a large amount of produced CO 2 with a selectivity of about 32% (Fig. 2e ). In stark contrast, Pd 1 /TiO 2 displays a very high C 2 H 6 production rate of ~0.91 mmol g –1 h –1 at the initial 1 h of light irradiation (Fig. 2d ). More importantly, catalyst stability has been dramatically improved (Supplementary Fig. 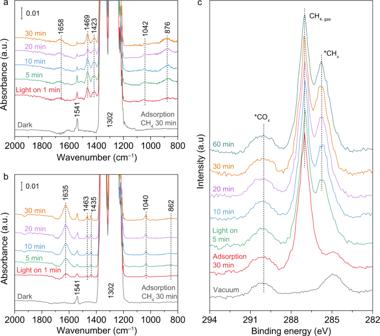Fig. 3: Intermediates detection for photocatalytic NOCM. a,bIn situ DRIFTS spectra for photocatalytic NOCM over Pd1/TiO2(a) and Pdn/TiO2(b).cIn situ high-resolution C 1 s XPS spectra of Pd1/TiO2catalyst with different light illumination time in 45 Pa CH4. 10 ), yielding C 2 H 6 at 2.6 mmol g –1 with over 93% carbon balance (Supplementary Table 3 ). The high C 2 H 6 production rate over Pd 1 /TiO 2 can be maintained with a 33-fold scale-up of catalyst usage under appropriate reaction conditions (Supplementary Fig. 11 ). These results clearly demonstrate that the modification of TiO 2 VBM with Pd SAs can allow the CH 4 conversion to proceed on the Pd instead of the lattice oxygen of TiO 2 , substantially suppressing overoxidation of CH 4 with lattice oxygen. As a direct outcome, the C 2 H 6 selectivity for Pd 1 /TiO 2 is maintained at ~94.3% (Fig. 2e ). Notably, we observe that the measured amount of produced H 2 is approximately in theoretically stoichiometric ratio with the production of C 2 H 6 and trace CO 2 (Supplementary Fig. 12 ), further confirming the superiority of Pd SAs in enhancing photocatalytic NOCM performance of TiO 2 . As a result, turnover number (TON) reaches as high as 186 toward C 2 H 6 evolution over the Pd 1 /TiO 2 catalyst for 3 h light irradiation. In terms of light utilization, the Pd 1 /TiO 2 catalyst achieves an AQE of 3.05% under 350-nm light irradiation (Fig. 2f ). Furthermore, the photocatalytic performance is directly proportional to the light intensity, demonstrating that the activation of CH 4 is driven by photogenerated holes under mild condition (Supplementary Fig. 13 ). The outstanding NOCM performance indicates that Pd SAs modification enables an efficient C–C coupling process and suppresses CH 4 overoxidation. To trace the origin of carbonaceous products, we further perform a series of control and isotope-labeling experiments (Supplementary Figs. 14 – 16 ), showing that the CH 4 is indeed the source of the produced C 2 H 6 . Insight into photocatalytic NOCM mechanism The information gleaned above has recognized the superior performance of CH 4 conversion by modifying VBM of TiO 2 with Pd SAs. We are now in a position to look into the reaction mechanism over TiO 2 with a focus on the role of Pd SAs. Based on photoelectrochemical measurements (Supplementary Fig. 17 ), it is demonstrated that the presence of Pd can greatly enhance the photogenerated charge carrier separation efficiency of the TiO 2 , and the Pd 1 /TiO 2 demonstrates the highest efficiency due to the homogeneous dispersion of Pd SAs on the TiO 2 . To gain insight into the intermediates of photocatalytic NOCM on Pd 1 /TiO 2 , electron paramagnetic resonance (EPR) measurement is performed to investigate possible radicals by using 5,5′-dimethyl-1-pyrroline N-oxide (DMPO) as a radical scavenger in a liquid-phase reaction condition [30] . As shown in Supplementary Fig. 18 , both the characteristic signals of ∙CH 3 and ∙OH can be detected using Pd 1 /TiO 2 . Given that the ∙OH is formed due to the presence of water, this observation indicates that the surface ∙CH 3 is the key intermediate for CH 4 coupling [31] , [32] . In comparison, only ∙OH is detected for pristine TiO 2 and Pd n /TiO 2 , suggesting the high efficiency of CH 4 dissociation on Pd 1 /TiO 2 . Furthermore, in situ diffuse reflectance-infrared Fourier-transform spectroscopy (DRIFTS) is employed to investigate the intermediates for photocatalytic NOCM. The catalysts are exposed to CH 4 under dark condition firstly for adsorption. As shown in Supplementary Fig. 19 , apart from the peak at 1302 cm –1 corresponding to C–H deformation vibration of CH 4 , the peak at 1541 cm –1 can ascribed to the symmetric deformation vibrational mode of CH 4 on metal oxide surface [17] , [33] . Upon light irradiation, the vibrational modes of CH 2 /CH 3 deformation at 1469 and 1423 cm –1 appear immediately (Fig. 3a ), indicating that CH 4 is rapidly dissociated over Pd 1 /TiO 2 surface by photogenerated charge carriers [8] . Furthermore, the peak of C–C stretching (876 cm –1 ) appears and gradually increase with the prolonged light irradiation, demonstrating C–C coupling on catalyst surface [8] , [34] . Meanwhile, the slight growth of C=O (1671 cm –1 ) and C–O (1042 cm –1 ) stretching vibrational modes are assigned to the species for CO 2 formation, suggesting the sluggish overoxidation of CH 4 on Pd 1 /TiO 2 [35] , [36] , [37] . In contrast, intense C=O and C–O stretching vibration signals can be observed for Pd n /TiO 2 (Fig. 3b ), while the CH 2 /CH 3 intermediates can hardly be resolved in the DRIFTS spectra for pristine TiO 2 (Supplementary Fig. 20 ). Taken together, photocatalytic NOCM results and in situ DRIFTS characterizations clearly reveal that Pd SAs modification can promote the coupling route and diminish the overoxidation of CH 4 under light irradiation. The surface hydrocarbon species are also monitored by in situ near ambient pressure XPS (NAP-XPS) studies. After introducing 45 Pa CH 4 into NAP-XPS chamber under the dark, the peak of gas-phase CH 4 (287.0 eV) is observed [38] . Subsequently, the peak of surface ∙CH x species at 285.6 eV appears and is gradually boosted along with light irradiation (Fig. 3c ), further corroborating the dissociation of CH 4 on catalyst surface [39] , [40] . Notably, the fitting curves of the C 1 s spectrum show the absence of C–O formation on the surface (Supplementary Fig. 21 ). This suggests that no C–O specie is involved in the CH 4 −to−C 2 H 6 conversion. Fig. 3: Intermediates detection for photocatalytic NOCM. a , b In situ DRIFTS spectra for photocatalytic NOCM over Pd 1 /TiO 2 ( a ) and Pd n /TiO 2 ( b ). c In situ high-resolution C 1 s XPS spectra of Pd 1 /TiO 2 catalyst with different light illumination time in 45 Pa CH 4 . Full size image To have a full image of the coupling process of NOCM, we perform DFT calculation to examine CH 4 dissociation and intermediate coupling over Pd 1 /TiO 2 with the assistance of photogenerated holes. In our calculation, Pd atom is stabilized in the fourfold hollow sites of TiO 2 (001) face to form Pd–O 4 complex. As demonstrated in our material screening, such a metal−support interaction modulates the VBM of TiO 2 . We, therefore, calculate the potential energy diagram of CH 4 coupling reaction on the Pd 1 /TiO 2 surface (Fig. 4a ), based on the atomic configurations in Fig. 4b . When CH 4 is adsorbed on Pd atom, the C–H bond is dissociated by the oxidation of photogenerated holes on Pd–O 4 unit, releasing H atom and leaving Pd–CH 3 (IM2) on the surface. Given the steric effect for adsorption, the activation of the second CH 4 requires a substantially higher energy of 1.35 eV (i.e., green line between IM3 and IM4). As a result, the extremely high activation energy of 1.74 eV (167.9 kJ mol –1 ) from initial state to TS state hinders the NOCM process under dark condition. However, taking the extra potential provided by the photogenerated holes into account (Supplementary Fig. 22 ), the energy barrier of the step turns into downhill (i.e., red line between IM3 to IM4), followed by the C–C coupling over Pd atom (TS to IM5) and C 2 H 6 desorption. Meanwhile, we also experimentally measure the activation energy of the NOCM process under light irradiation condition. A relatively low value of 9.54 kJ mol –1 is acquired (Supplementary Fig. 23 ). The dramatic decrease of activation energy under light irradiation suggests that the photogenerated carriers play a crucial role in overcoming the energy barrier of NOCM. Nevertheless, the simulation suggests that the efficiency of C–C coupling should be associated with the probability of the second CH 4 reaching the active site, depending on the concentration of gaseous CH 4 . In our photocatalytic tests, we indeed recognize that the yield of C 2 H 6 decreases when reducing the concentration of filling CH 4 (Supplementary Fig. 24 ). Fig. 4: DFT calculations for photocatalytic NOCM. a Free-energy diagrams for C 2 H 6 production on Pd 1 /TiO 2 with hole energy ( U h ) of 0 eV and 2.85 eV. b Atomic configurations for the corresponding steps in the simulation. Full size image Performance enhancement with lattice oxygen stabilization As revealed by the photocatalytic NOCM, the C 2 H 6 is the primary product along with the minor CO 2 using Pd 1 /TiO 2 . Note that no gaseous oxygen or other oxidizing agent is present in the reactor, implying that the overoxidation of CH 4 to CO 2 is derived from lattice oxygen of the catalyst [15] , [16] , [17] , [18] . Such oxidation by lattice oxygen is inevitably accompanied with its consumption that will eventually reduce photocatalytic performance. To this end, we investigate the time-dependent NOCM on Pd 1 /TiO 2 (Supplementary Figs. 25 and 26 ), showing that the performance of the Pd 1 /TiO 2 decays after 6 h of reaction and can be recovered by heating the catalyst in air. As such, the photocatalytic performance of Pd 1 /TiO 2 is well maintained for eight cyclic tests with each cycle of 3 h followed by a recovering process (Fig. 5a ). Furthermore, the characterizations including aberration-corrected HAADF-STEM, CO adsorption DRIFTS and EXAFS for Pd 1 /TiO 2 after the cyclic tests show the chemical state of Pd is well preserved with single dispersion (Supplementary Figs. 27 − 29 ). Moreover, the H 2 –temperature-programmed reduction (H 2 –TPR) analysis shows that the Pd–O species in Pd 1 /TiO 2 are more stable than Pd oxide, indicating the stability of Pd–O 4 units (Supplementary Fig. 30 ). Apparently, the overoxidation of CH 4 to CO 2 can be suppressed by Pd 1 /TiO 2 through the contribution of Pd SAs to VBM but still occurs via the consumption of lattice oxygen. On the basis of DFT calculation (Fig. 4b , IM2), we can elucidate the mechanism for the consumption of lattice oxygen on Pd 1 /TiO 2 that one of Pd–O bonds in Pd–O 4 unit is fractured to steady the state of [Pd…∙CH 3 ] after CH 4 activation on the Pd atom. As such, the exposed O atom from the fractured Pd–O, together with other O atoms uncoordinated with Pd atoms, can be consumed to produce CO 2 via overoxidation, resulting in performance decay. Fig. 5: Evidence and prevention strategy for lattice oxygen consumption. a Production rates and selectivity of C 2 H 6 in the cyclic tests by Pd 1 /TiO 2 . Each cycle lasts 3 h, between which the catalyst is treated in air. b In situ EPR signals for Pd 1 /TiO 2 catalyst in 0.1 MPa CH 4 under different conditions. The inset is the formation of O vacancy during the reaction. c In situ high-resolution O 1 s XPS spectra for Pd 1 /TiO 2 catalyst with different light illumination time in 45 Pa CH 4 . d , e The comparison of C 2 H 6 ( d ) and CO 2 ( e ) production between Pd 1 /TiO 2 and Pd 1 /ST. f The photocatalytic NOCM by Pd 1 /ST and Pd 1 /TiO 2 benchmarked against the photocatalytic NOCM and the mild-condition thermocatalytic NOCM in literature. The temperatures in thermocatalysis represent the reaction temperatures applied in those works. Full size image To further prove the mechanism, we employ in situ EPR to examine the structural changes of the catalysts during photocatalytic NOCM. Upon light irradiation, Pd 1 /TiO 2 shows the signal for −O •– radical sites in anatase crystals at g = 1.999, which is derived from the separation of photogenerated charge carriers and can participate in CH 4 oxidation (Fig. 5b ) [41] . After turning light off, the signal for the single electron trapped O defects at g = 2.001 can be observed, manifesting the emergence of O vacancies after the photocatalytic process [42] . A similar observation is also acquired for pristine TiO 2 (Supplementary Fig. 31 ). Furthermore, the appearance of the O vacancy during the reaction can be further attested via the in situ NAP-XPS, corresponding with the results of in situ EPR (Fig. 5c , Supplementary Figs. 32 and 33 ) [23] , [43] . As determined by temperature-programmed oxidation (TPO), 0.7 wt.% of lattice oxygen has been consumed in the photocatalytic process (Supplementary Fig. 34 ). Moreover, the location of the formed O vacancies is determined by 17 O magic angle spinning nuclear magnetic resonance ( 17 O MAS NMR) and EPR spectra. It turns out that the consumption of lattice oxygen preferentially takes place at the O atoms near the Ti sites with 2-fold oxide coordination (OTi 2 ) on the catalyst surface (Supplementary Fig. 35 ). Given the experimental results indicating the CH 4 overoxidation process, we further conduct DFT calculation to simulate the possible steps of CH 4 –to–CO 2 conversion with lattice oxygen consumption. As shown in Supplementary Fig. 36 , taking the O site adjacent to Ti atom as an example, the photogenerated holes are required to provide extra potential for CH 4 dehydrogenation at the O site; otherwise, the high energy barrier of further steps will inhibit the process thermodynamically. Specifically, the activation of the last hydrogen atom in CH 4 requires a high energy of 1.82 eV (i.e., green line between O-IM4 and O-IM5), which is the rate-determining step for overoxidation process under dark condition. However, the energy barrier of this step turns into downhill with the assistance of photogenerated holes (i.e., red line between O-IM4 and O-IM5), and the bonding between the adsorbed CH 4 and the second lattice oxygen becomes the rate-determining step with the energy barrier of 1.12 eV (i.e., O-IM3 to O-IM4). This indicates that the stabilization of the lattice oxygen can weaken the bonding between CH 4 and O site and suppress the overoxidation of CH 4 to CO 2 under light irradiation. The mechanistic study suggests that the stabilization of lattice oxygen should be an efficient method for further suppressing the CH 4 overoxidation and enhancing the stability of Pd 1 /TiO 2 . To this end, we employ the elemental doping via Si to further stabilize O atoms of TiO 2 (Supplementary Fig. 37 ) [44] . As shown in Fig. 5d as well as Supplementary Figs. 38 and 39 , incorporating Si into Pd 1 /TiO 2 (Pd 1 /ST) can mitigate CH 4 overoxidation to a large extent and maintain photocatalytic activity for up to 24 h. The effect of Si doping on suppressing CH 4 overoxidation is further verified by the comparison of CO 2 production between Pd 1 /TiO 2 and Pd 1 /ST (Fig. 5e ). Moreover, the computational results demonstrate that the incorporation of Si can further increase the energy barrier of the rate-determining step in the conversion process of CH 4 to CO 2 as compared with that of Pd 1 /TiO 2 , indicating that the presence of Si atoms in TiO 2 can suppress the overoxidation of CH 4 by stabilizing the lattice oxygen atoms (Supplementary Fig. 40 ). It is worthwhile to note that the photocatalytic performance of optimized Pd 1 /TiO 2 and Pd 1 /ST well exceed the existing photocatalysts for NOCM and reach the level of thermocatalysts working between 923 and 1073 K (Fig. 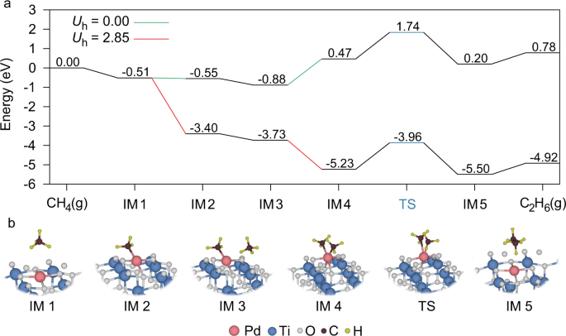Fig. 4: DFT calculations for photocatalytic NOCM. aFree-energy diagrams for C2H6production on Pd1/TiO2with hole energy (Uh) of 0 eV and 2.85 eV.bAtomic configurations for the corresponding steps in the simulation. 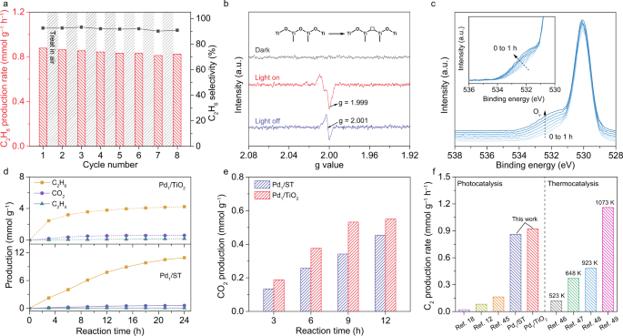Fig. 5: Evidence and prevention strategy for lattice oxygen consumption. aProduction rates and selectivity of C2H6in the cyclic tests by Pd1/TiO2. Each cycle lasts 3 h, between which the catalyst is treated in air.bIn situ EPR signals for Pd1/TiO2catalyst in 0.1 MPa CH4under different conditions. The inset is the formation of O vacancy during the reaction.cIn situ high-resolution O 1 s XPS spectra for Pd1/TiO2catalyst with different light illumination time in 45 Pa CH4.d,eThe comparison of C2H6(d) and CO2(e) production between Pd1/TiO2and Pd1/ST.fThe photocatalytic NOCM by Pd1/ST and Pd1/TiO2benchmarked against the photocatalytic NOCM and the mild-condition thermocatalytic NOCM in literature. The temperatures in thermocatalysis represent the reaction temperatures applied in those works. 5f and Supplementary Table 4 ) [45] , [46] , [47] , [48] , [49] . To address the limitations in photocatalytic NOCM, we have developed a photocatalyst based on TiO 2 by modifying valence band near-surface with Pd – O 4 units, which achieves highly efficient light-driven CH 4 conversion to C 2 H 6 under mild condition. Benefiting from the contribution of Pd – O 4 units to valence band, the single Pd sites display the accumulation of photogenerated holes, which are able to dissociate C–H bond and adsorb ∙CH 3 for C 2 H 6 formation. In the meantime, reducing the role of O atoms in valence band substantially suppresses the overoxidation of CH 4 with lattice oxygen, dramatically improving catalytic durability. As a result, the catalyst exhibits the ultrahigh C 2 H 6 production rate of 0.91 mmol g –1 h –1 and selectivity of 94.3%, reaching the level of thermocatalytic NOCM at relatively mild condition. Fundamentally, the in situ generation and retention of O vacancies on photocatalysts during photocatalytic NOCM have been experimentally observed and assigned to the consumption of lattice oxygen for CO 2 generation, providing key information for further performance enhancement. Interestingly, the overoxidation process can be suppressed by steadying subsurface lattice oxygen with lattice doping, further enhancing catalyst reusability. This work highlights the importance of rational lattice engineering to tuning reaction pathways, and is expected to offer guideline for the design of high-performance catalysts toward NOCM at mild condition. Catalysts preparation TiO 2 nanosheets were prepared by a simple hydrothermal method. Typically, 10 mL of tetrabutyl titanate (TBOT) was mixed with 1.6 mL HF with stirring for 30 min. Then the solution was transferred into a 50 mL Teflon-lined autoclave and reaction at 180 °C for 24 h. After that, the resulting white slurry was centrifuged and washed with distilled water several times and dried in a vacuum oven. For the synthesis of Pd 1 /TiO 2 catalyst, 20 mg TiO 2 nanosheets were dispersed in 5 mL dilute ammonia solution (pH = 10.5) to form a homogeneous white suspension. Separately, 20 μL Pd(NO 3 ) 2 solution (21.1 mM) was attenuated with dilute ammonia solution (pH =  10.5) to 3 mL. Next, the 3 mL mixture was injected into the TiO 2 suspension with stirring by using the syringe pump at a rate of 1 mL h –1 , followed by vigorous stirring for another 3.5 h. The obtained slurry was then washed with distilled water until the pH turns neutral and dried in the oven at 60 °C. After that, the collected solid was calcined in air at 300 °C in air for 2 h. The Pd n /TiO 2 was prepared by reduction of NaBH 4 . Generally, 60 mg of TiO 2 nanosheets were dispersed in 30 mL distilled water, then 60 μL Pd(NO 3 ) 2 solution (21.1 mM) was added into the mixture and further react with 5 mg NaBH 4 . The product was separated by centrifugation, washed with water several times and dried in a vacuum oven at 60 °C overnight. The other metal SAs loaded M 1 /TiO 2 catalysts were synthesized with the similar electrostatic adsorption wet impregnation technique by adding different metallic precursor solution with approximate content. For Si-doping TiO 2 , 150 μL Tetraethoxysilane, 10 mL TBOT, and 1.2 mL HF were added into anhydrous ethanol (20 mL) with stirring for 30 min. The precursor solution was transferred into 50 mL Teflon-lined autoclave and reaction at 180 °C for 2 h. The Pd 1 /ST was obtained by a similar procedure with Pd 1 /TiO 2 . Characterization Powder X-ray diffraction patterns were recorded by using a Philips X’Pert Pro Super X-ray diffractometer with Cu–Kα radiation ( λ = 1.54178 Å). Transmission electron microscopy (TEM) images were taken on a Hitachi Model H-7700 microscope at 100 kV. High-resolution TEM (HRTEM) images were taken on a JEOL JEM-2100 field-emission higher-resolution transmission electron microscope at 200 kV. The aberration-corrected HAADF-STEM images and corresponding EDS mapping profiles were measured on the JEOL ARM-200F field-emission transmission electron microscope operated at 200 kV. UV-Vis diffuse reflectance data were recorded in the spectral region of 200–800 nm with a Shimadzu SolidSpec-3700 spectrophotometer. The X-ray adsorption fine structure (XAFS) spectra of sample were acquired at beamline 1W1B of the Beijing Synchrotron Radiation Facility (BSRF) and beamline 14W1 of the Shanghai Synchrotron Radiation Facility (SSRF). For XANES spectra, the experimental absorption coefficients as a function of energies were processed by background subtraction and normalization procedures and reported as the normalized intensity. The acquired EXAFS data were processed according to the standard procedure using the WinXAS3.1 program. The in situ NAP-XPS measurements were carried at the beamline BL02B1 of SSRF under light irradiation (365 nm LED light) or dark condition. In situ EPR spectra for oxygen vacancies detection are obtained on the JEOL JES-FA200 spectrometer equipped with a 500 W xenon lamp as the illumination source. Detection of methyl radical (∙CH 3 ) 5, 5'-dimethyl-1-pyrroline N-oxide (DMPO) was used to trap the generated methyl or hydroxyl radicals in the reaction system. Briefly, the as-prepared catalysts and DMPO are dispersed in ice-bath DI water. The mixture was vigorously shaken for 10 s and irradiated under 0.1 MPa CH 4 by using a 500 W xenon lamp, and then analyzed by EPR spectroscopy. DRIFTS for CO adsorption DRIFTS measurements were performed using a Bruker IFS 66 v Fourier-transform spectrometer equipped with Harrick diffuse reflectance accessory with ZnSe and quartz window at BL01B in the National Synchrotron Radiation Laboratory (NSRL) in Hefei, China. After the sample was loaded into the reaction chamber, pure Ar (99.999%) was purged into the chamber firstly for background spectra collection. Subsequently, CO was introduced into the system until CO adsorbed saturation. Then the pure Ar was purged to remove the gaseous CO and the spectra were collected by averaging 128 scans at a resolution of 2 cm –1 . In situ DRIFTS for CH 4 activation In situ DRIFTS measurements were performed using a Bruker IFS 66 v Fourier-transform spectrometer equipped with Harrick diffuse reflectance accessory with ZnSe and quartz window at BL01B in the NSRL in Hefei, China. Each spectrum is recorded by averaging 128 scans at a resolution of 2 cm –1 . After sample loading, the pure Ar was purged into the chamber for background spectra collection. Subsequently, pure CH 4 (99.999%) is introduced into the chamber for 10 min. For CH 4 -adsorption process, the spectra were collected under dark condition at 5, 10, 20, and 30 min, respectively. After that, the system was exposed to light irradiation and the spectra were collected when the irradiation times are 1, 5, 10, 20, and 30 min, respectively. Photocatalytic CH 4 conversion measurements The photocatalytic CH 4 conversion experiments were carried out in CH 4 atmosphere (0.1 MPa) at room temperature in a 30 mL custom-made quartz tube reactor. In a typical test, 3.0 mg of catalyst is dispersed in 800 μL of DI water and then dropped onto a 1 × 3 cm clear glass and dried in air at 323 K. After the glass was vertically placed in the reactor, 1 vol %, 10 vol % CH 4 /Ar or pure CH 4 was purged into the system. The reactor was irradiated by a 300 W xenon lamp (PLS-SXE300, Perfect light). The produced H 2 and hydrocarbons were quantified by a gas chromatograph (GC, 7890B, Ar carrier, Agilent) equipped with thermal conductivity detector (TCD) and flame ionization detector (FID). Another GC (Techcomp GC-7900, China) equipped with a TDX-01 packed column was employed to determine the amounts of CO and CO 2 . The isotope-labeled experiments were performed by using pure 13 CH 4 , 12 CH 4 , or CD 4 as feeding gas. The products were analyzed with gas chromatography-mass spectrometry (GC–MS, 7890 A and 5975 C, He carrier, Agilent). For the regeneration treatment, the catalyst was heated under 80 °C for 2 h in air. Determination of AQE for C 2 H 6 production The AQE was obtained by using different monochromatic filters (350, 380, 400, 450, 500, and 600 nm) during light irradiation. The irradiance values in ultraviolet region were measured by an UV energy meter (UV DESIGN, UV-int 140). The AQE was calculated through the following equation: 
    AQE=N_e/N_p=n× M×N_A/W× S× t/h× v× 100 %
 (1) where N e and N p represent the number of reacted electrons and incident photons, respectively, n is the number of electrons transferred during C 2 H 6 formation, M is the molar number of C 2 H 6 , N A is the Avogadro’s constant, and W , S , t , h , and v are the light intensity, irradiation area, irradiation time, Planck constant and light frequency, respectively. Photocurrent measurements The photoelectrochemical measurements were performed on CHI 660E electrochemical workstation (CH Instruments) in three-electrode system under light irradiation. In all, 3.0 mg of catalyst was dispersed in 800 μL of DI water and then dropped onto a 1 × 3 cm fluorine-doped tin oxide (FTO)-coated glass for employed as work electrode. The Pt foil and saturated Ag/AgCl electrode were used as counter electrode and reference electrode, respectively. 0.5 M Na 2 SO 4 aqueous solution was chosen as the electrolyte. The electrolyte was saturated with pure Ar or CH 4 prior before the tests. The photocurrent responses of the prepared photoelectrodes (i.e., I–t) were operated by measuring the photocurrent densities under chopped light irradiation (light on/off cycles: 50 s) at a bias potential of 0.8 V vs. Ag/AgCl for 800 s. Calculation of carbon balance Carbon balance was calculated through the following equation: 
    Carbon  balance=Moles of products in terms of carbon/Moles of methane consumed× 100 %
 (2) Computational method The spin-polarized density functional theory (DFT) calculations were performed by using the Vienna ab initio simulation package (VASP) [50] , [51] . The interaction between the core and valence electrons was described using the frozen-core projector augmented wave (PAW) approach [52] , [53] . The generalized gradient approximation of Perdew–Burke–Ernzerhof (PBE) functional was used [54] . The energy cutoff was set to be 400 eV. The DFT-D2 vdW correction proposed by Grimme was adopted to describe long-range vdW interactions [55] . The convergence criteria of energy and force were set to be 10 −5 eV and 0.02 eV Å −1 , respectively. A Monkhorst–Pack grid of 9 × 9 × 3 k-points was used to sample the Brillouin zone of the unit cell for the anatase TiO 2 . The optimized lattice parameters were a = b = 3.789 Å and c = 9.479 Å. A 3 × 3 supercell with five layers of TiO 2 was used to describe the (001) surface. The bottom layer Ti and O dangling bonds were saturated with pseudo-hydrogens with nuclear charges of +1.25 and +0.75, which has been reported in previous studies [56] , [57] . A vacuum space greater than 15 Å perpendicular to the surface was applied to separate the interactions between neighboring slabs. The Brillouin zone was sampled by the 1 × 1 × 1 Γ -centered k-point for the slab system. The energy differences (Δ E ) for the reactions were calculated according to the approach originally proposed by Nørskov and coworkers [58] , [59] , Δ E = Δ E 0 + Δ E U , where Δ E 0 is the computed reaction energy. The external potential supplied by photogenerated holes was added by Δ E U = −e U h , where U h is the electrode potential relative to the standard hydrogen electrode (SHE). The transition states were searched with the nudged elastic band method with climbing images [60] .